Formation of lunar swirls by magnetic field standoff of the solar wind Lunar swirls are high-albedo markings on the Moon that occur in both mare and highland terrains; their origin remains a point of contention. Here, we use data from the Lunar Reconnaissance Orbiter Diviner Lunar Radiometer to support the hypothesis that the swirls are formed as a result of deflection of the solar wind by local magnetic fields. Thermal infrared data from this instrument display an anomaly in the position of the silicate Christiansen Feature consistent with reduced space weathering. These data also show that swirl regions are not thermophysically anomalous, which strongly constrains their formation mechanism. The results of this study indicate that either solar wind sputtering and implantation are more important than micrometeoroid bombardment in the space-weathering process, or that micrometeoroid bombardment is a necessary but not sufficient process in space weathering, which occurs on airless bodies throughout the solar system. Lunar swirls have been documented since the Apollo era [1] , and since that time, a variety of swirl morphologies has been identified, ranging from the complex structures present in the Reiner Gamma formation, Mare Ingenii and Mare Marginis swirls, to simple bright patches with diffuse edges, as at Descartes. Intermediate morphologies occur near Airy and Gerasimovich craters [2] . Several swirl formation mechanisms have been proposed, including (1) solar wind standoff due to the presence of local magnetic fields, preventing solar wind sputtering and implantation, nanophase iron formation, and the resulting surface darkening associated with space weathering [3] , (2) recent comet impacts or micrometeoroid swarms that scoured the lunar surface, leaving a fine-gained, unweathered material and possibly imparting a remnant magnetization [4] , [5] , [6] , and (3) electrostatic levitation and deposition of high-albedo, fine-grained, feldspar-enriched dust [7] . The association of all swirls with magnetic field anomalies of varying strength [8] , [9] , [10] has driven the development of each of these hypotheses. In this work, we use the unique mid-infrared data set from the Diviner Lunar Radiometer to distinguish between these hypotheses. We show that Diviner data support the solar wind standoff model for lunar swirl formation and disqualify the impact swarm and dust transport hypotheses. Previous near-infrared observations of lunar swirls show them to be optically immature compared with the surrounding terrains [10] . Space weathering leads to optical maturation of the surfaces of airless bodies and is thought to be caused by two main processes: (1) solar wind sputtering and/or implantation of hydrogen atoms, leading to the formation of nanophase metallic iron blebs and (2) micrometeoroid bombardment that leads to the formation of agglutinitic glass and a reduced vapour-deposited coating [11] . Under the solar wind standoff model, horizontal magnetic fields at the lunar swirl sites deflect the solar wind, preventing most sputtering and implantation of solar wind ions [12] , [13] . If this is the case, micrometeoroid bombardment should be the major relevant space-weathering process [14] at swirl sites. A relative lack of solar wind interaction with the lunar surface at swirl sites is supported by recent observations from the Moon Mineralogy Mapper (M 3 ) instrument that confirm the Clementine observations of a substantial reduction in optical maturity and also show a reduction of the presence of surface hydroxyls at the swirl sites [15] . Recent observations in the ultraviolet by the Lunar Reconnaissance Orbiter Camera Wide Angle Camera subsystem also suggest that micrometeoroid bombardment, and not solar wind interaction, plays the dominant role in space weathering at the lunar swirls [16] . Diviner has three narrow band infrared channels near 8 μm, from which the silicate Christiansen Feature (CF) can be calculated [17] . The position of the CF is related to the degree of mineral silicate polymerization and provides an indicator of composition [18] . However, analysis of the global observations by Diviner has revealed that the CF position is also influenced by optical maturity. Optically mature surfaces are shifted to longer wavelengths by~0.1 μm (or about ~20% of the full range of lunar CF values that have been measured) compared with immature surfaces with the same composition [19] . A global CF map [19] shows substantial anomalies related to young, fresh craters such as Tycho and Jackson, which have CF positions at shorter wavelengths than the surrounding mature terrain. Here we find that Diviner data show the CF anomalies are due to abnormal space weathering at both the mare and highland swirl sites. This result, in addition to the relative lack of thermophysical anomalies at the swirl sites, strongly supports the solar wind standoff model and disqualifies the micrometeoroid/comet swarm and dust levitation models for swirl formation. Diviner data can be used to determine the composition and degree of space weathering of the lunar surface [17] , [19] , [20] and to determine thermophysical properties using daytime and night-time thermal infrared measurements [21] , [22] . The ability to characterize both the compositional and thermophysical properties of the lunar regolith make Diviner well suited to examine the swirls and differentiate between the three proposed formation mechanisms. 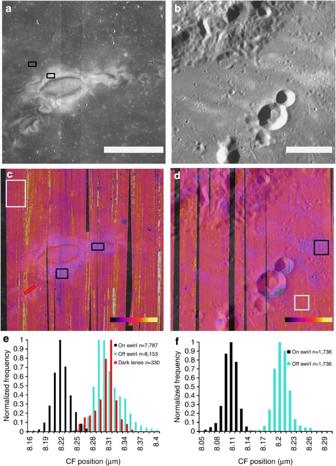Figure 1: Diviner CF position data for the Reiner Gamma and Van de Graaff crater swirls. (a) Wide Angle Camera (WAC) base map for Reiner Gamma. Black boxes indicate the regions used for surface roughness and thermal model analysis inFigs 5and8. Scale bar, 50 km. (b) WAC base map for Van de Graaff crater. Scale bar, 20 km. (c) CF position map of the Reiner Gamma swirl stretched from 8.15 to 8.45 μm overlayed on Lunar Reconnaissance Orbiter Camera (LROC) WAC mosaic. (d) CF position map of the Van de Graaff crater swirls stretched from 8.0 to 8.4 μm overlayed on LROC WAC mosaic. (e) Normalized histogram of CF values on the Reiner Gamma swirl (black boxes inc), off the swirl (white box in1c), and in the dark lanes (yellow boxes inc). (f) Normalized histogram of CF values on the Van de Graaff crater swirls (black box inb) and off the swirl (white box in1b). Diviner CF anomaly at swirl sites We analysed Diviner data covering 12 swirl regions including both the mare and highlands sites ( Figs 1 and 2 ; Table 1 , Supplementary Figs 1–10 ). At both the Reiner Gamma and Van de Graaff crater sites, the distributions of CF values on and off the swirls are clearly separated. Garrick-Bethell et al . [7] demonstrated that only a small portion of the Reiner Gamma ‘dark lanes’ (small curvilinear low-albedo regions that occur between some high-albedo swirls) are truly darker than the surrounding terrain at visible wavelengths. We found that the CF distribution of this portion of the dark lanes within Reiner Gamma is nearly identical to the off-swirl distributions ( Fig. 1 ). The off-swirl locations were defined to be well outside the visible light albedo boundaries of the swirls identified in Lunar Reconnaissance Orbiter Camera wide angle camera or Clementine data. The average off-swirl CF values at Reiner Gamma (8.31 μm) and Van de Graaff (8.20 μm) are close to the previously determined global average mare and highland CF values [17] . The average on-swirl values for Reiner Gamma and Van de Graaff are shifted to shorter wavelengths by 0.08 and 0.09 μm, respectively. In addition, three-point Diviner spectra acquired both on and off the swirls at both the sites show clear differences in the spectral shape, which is reflected in the differences in modelled CF values for these sites. Swirl spectra were acquired from the regions outlined by boxes in Fig. 1 and the average spectra and resulting modelled CF values are shown in Fig. 2 . Figure 1: Diviner CF position data for the Reiner Gamma and Van de Graaff crater swirls. ( a ) Wide Angle Camera (WAC) base map for Reiner Gamma. Black boxes indicate the regions used for surface roughness and thermal model analysis in Figs 5 and 8 . Scale bar, 50 km. ( b ) WAC base map for Van de Graaff crater. Scale bar, 20 km. ( c ) CF position map of the Reiner Gamma swirl stretched from 8.15 to 8.45 μm overlayed on Lunar Reconnaissance Orbiter Camera (LROC) WAC mosaic. ( d ) CF position map of the Van de Graaff crater swirls stretched from 8.0 to 8.4 μm overlayed on LROC WAC mosaic. ( e ) Normalized histogram of CF values on the Reiner Gamma swirl (black boxes in c ), off the swirl (white box in 1c ), and in the dark lanes (yellow boxes in c ). ( f ) Normalized histogram of CF values on the Van de Graaff crater swirls (black box in b ) and off the swirl (white box in 1b ). 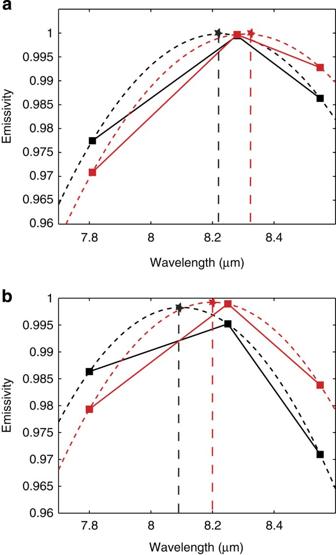Figure 2: Average Diviner spectra. Spectra are averaged using data from the white and black boxes outlined inFig. 1. (a) Reiner Gamma swirl. (b) Van de Graaff crater swirl. Black spectra are average on-swirl spectra. Red spectra are average off-swirl spectra from the boxes outlined inFig. 1. The parabolic traces represent the fitting function used to determine the CF position (stars) from the spectra. Full size image Figure 2: Average Diviner spectra. Spectra are averaged using data from the white and black boxes outlined in Fig. 1 . ( a ) Reiner Gamma swirl. ( b ) Van de Graaff crater swirl. Black spectra are average on-swirl spectra. Red spectra are average off-swirl spectra from the boxes outlined in Fig. 1 . The parabolic traces represent the fitting function used to determine the CF position (stars) from the spectra. Full size image Table 1 CF and OMAT parameter values for each swirl examined in this study. Full size table The low CF position values of each of the swirls are clearly associated with lower optical maturity compared with the surrounding terrains ( Table 1 ). 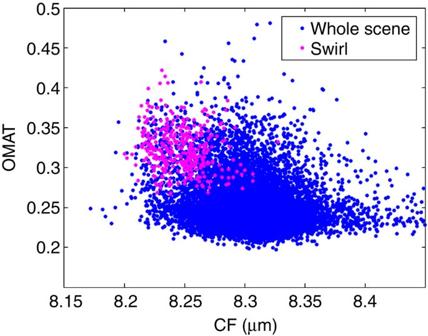Figure 3: Comparison of CF position and OMAT maturity index for Reiner Gamma. On-swirl pixels (taken from the regions outlined by white boxes inFig. 1) clearly have lower CF and higher OMAT (lower maturity) values than the median scene. Figure 3 shows the relationship between CF position and the optical maturity parameter (OMAT) [23] derived from Clementine multispectral data at Reiner Gamma. Compared with the scene average, swirl pixels have both lower overall CF and higher OMAT (lower maturity) values. Figure 3: Comparison of CF position and OMAT maturity index for Reiner Gamma. On-swirl pixels (taken from the regions outlined by white boxes in Fig. 1 ) clearly have lower CF and higher OMAT (lower maturity) values than the median scene. Full size image At Reiner Gamma, Airy, Firsov and Rima Sirsalis, the complex swirls have easily identifiable dark lanes between the high-albedo regions. At Airy, the background terrain albedo varies substantially, so it is difficult to determine if the dark lanes are, in fact, lower albedo than the surrounding terrain. However, at Firsov and Rima Sirsalis, the dark lanes ( Fig. 4a,b ) have demonstrably lower visible albedos than the surrounding terrain. In Fig. 4c,d , we plot the Clementine 950-nm/750-nm reflectance ratio against the 750-nm ratio for regions on the swirl, in the dark lanes, and on the local surrounding terrain. The dark lanes at these sites are the darkest sampled regions in the scene. At these sites, the averages and distributions of the CF values just off the swirls and within the dark lanes of each swirl are within 0.01 μm, and dark lane OMAT values are nearly identical to the surrounding terrain ( Table 1 ). These data are consistent with the hypothesis that magnetic field lines over the dark lanes have a vertical orientation, allowing the solar wind to interact with the surface [24] . It has previously been suggested that the dark lanes and low-albedo off-swirl regions associated with some swirls result from an increased rate of space weathering as the charged solar wind particles deflected by local magnetic fields are funneled to these regions [14] . However, maturity enhancements in the dark lanes are not detected in Diviner data. Rather, the nearly identical CF distributions within the dark lanes and the local terrains near the swirls (for example, Fig. 1 ) suggest that the main effects of space weathering at mid-infrared wavelengths (shift in CF position to longer wavelengths) reach a maximum early in the space-weathering process and are not enhanced on increased flux of solar wind particles. 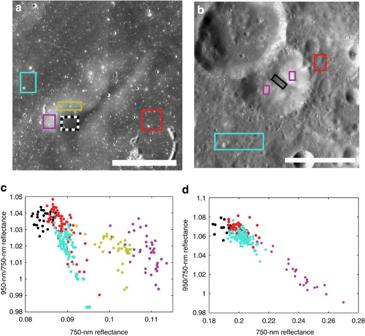Figure 4: Clementine albedo variations associated with swirl dark lanes. Dark lanes at Rima Sirsalis and Firsov crater have lower visible albedos than surrounding terrain. (a) Rima Sirsalis 750-nm reflectance. Scale bar, 25 km. (b) Firsov crater 750-nm reflectance. Scale bar, 25 km. (c) Rima Sirsalis 950/750-nm reflectance ratio versus 750-nm reflectance. Coloured points correspond to the coloured boxes ina. Black dots correspond to the white dotted box ina. (d) Firsov crater 950/750-nm reflectance ratio versus 750-nm reflectance. Coloured points correspond to the coloured boxes inb. Figure 4: Clementine albedo variations associated with swirl dark lanes. Dark lanes at Rima Sirsalis and Firsov crater have lower visible albedos than surrounding terrain. ( a ) Rima Sirsalis 750-nm reflectance. Scale bar, 25 km. ( b ) Firsov crater 750-nm reflectance. Scale bar, 25 km. ( c ) Rima Sirsalis 950/750-nm reflectance ratio versus 750-nm reflectance. Coloured points correspond to the coloured boxes in a . Black dots correspond to the white dotted box in a . ( d ) Firsov crater 950/750-nm reflectance ratio versus 750-nm reflectance. Coloured points correspond to the coloured boxes in b . Full size image The dust levitation model of lunar swirl formation [7] suggests that the spectral character of the swirls should be affected by a minor addition of feldspar, which is slightly enriched in the finest size fraction of the lunar soil [25] . Detailed analyses of the modal abundances of major minerals in sieved fractions of lunar soils show that feldspar is typically enriched by ~2–4 wt. % compared with coarser size fractions [26] . Therefore, the dust levitation model suggests an enrichment of feldspar in the optically active surface layer of mare swirls by a comparable amount, assuming that all of the levitated dust is<10 μm in diameter. Laboratory spectroscopic measurements of olivine-feldspar mixtures in a simulated lunar environment [27] ( Fig. 5 ) show that ~16 wt.% feldspar would need to be added to account for a typical mare swirl CF shift from ~8.3 to ~8.2 μm. At the highlands sites,~20 wt.% feldspar would need to be added to the swirl sites to account for a CF shift from ~8.2 to ~8.1 μm. While it is a simplification to model the swirl sites as olivine-feldspar mixtures, the laboratory data do suggest that the required feldspar contributions to the swirl CF shifts are ~5 to 10 times higher than the levels predicted by the dust levitation model. Swirls in both the highlands and mare consistently show CF shifts of ~0.04 to 0.09 μm to shorter wavelengths. Rather than an addition of a small amount of feldspar, this shift is comparable to CF shifts attributed to the optically immature surfaces. The Diviner data, therefore, suggest that a layer of fine particulate feldspar-enriched material is not responsible for the lunar swirl albedo anomalies and spectral properties. This interpretation supports visible and near-infrared measurements from the M 3 instrument [15] . 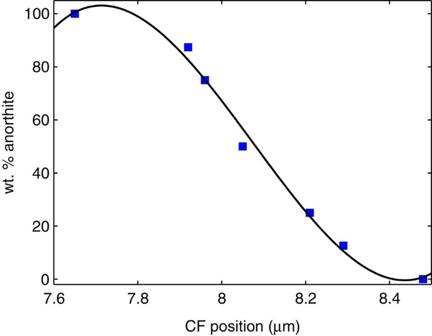Figure 5: CF positions of olivine-plagioclase mixture spectra acquired in a simulated lunar environment. Regression of the data using a degree 3 polynomial shows that to go from a CF of 8.3 to 8.2 μm, ~16 wt.% additional feldspar needs to be added to the mixture. To go from 8.2 to 8.1 μm, ~20 wt. % additional feldspar must be added. Figure 5: CF positions of olivine-plagioclase mixture spectra acquired in a simulated lunar environment. Regression of the data using a degree 3 polynomial shows that to go from a CF of 8.3 to 8.2 μm, ~16 wt.% additional feldspar needs to be added to the mixture. To go from 8.2 to 8.1 μm, ~20 wt. % additional feldspar must be added. Full size image Surface roughness at swirl sites In addition to compositional analysis, we can use the daytime Diviner data to address the physical state of the lunar surface. We employ a roughness model [28] ( Fig. 6 ) and Diviner daytime measurements in channels 3 and 6 (12.5–25 μm) to determine the spectral aniosthermality caused by surface roughness at Reiner Gamma. Surface roughness varies with length scale, and becomes greater with decreasing scale [29] . Previous lunar surface roughness estimates have included Lunar Orbiter Laser Altimeter data at metre to decametre scales [30] , visible photometric studies typically at sub-mm scales [31] , [32] and additional sub-mm surface roughness estimates from in situ high-resolution imagery [29] . At sub-mm to cm scales, typical lunar surface roughness values, defined as a root mean square (RMS) slope are 16–25° (ref. 29 ). Previous thermal infrared observations of the Moon and Mars have shown substantial effects due to surface roughness at ~cm scales [33] , [34] , [35] , [36] , [37] . Diviner data offer the ability to characterize cm-scale surface roughness at the high spatial resolution (128–256 ppd (pixels per degree)) typical of the instrument. 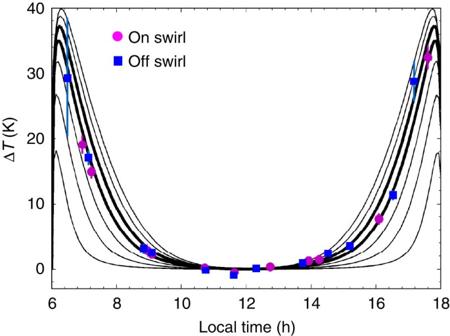Figure 6: Reiner Gamma roughness model. Modelled brightness temperature deviations between the channels 3 and 6 as function of the local time are plotted for RMS surface slopes varying in 5° increments from 10° (bottom line) to 40° (top line). Measured data from the Reiner Gamma swirl are displayed as magenta circles. Data from a nearby off-swirl surface are displayed as blue squares. Error bars are 1 s.d. Curves representing 25–30° roughness are bold. Diviner data from Reiner Gamma swirl indicate surface roughness in this range. Figure 6 shows the modelled change in the channel 3−channel 6 brightness temperature differences (ΔBT) on and off the Reiner Gamma swirl as a function of time of day for different RMS surface slope along with ΔBT data from 6 am to 6 pm local time. Within a standard deviation of the temperature measurements, Diviner data indicate nearly identical surface roughnesses of~25–30° both on and off the swirl (bold curves in Fig. 6 ). This surface roughness reflects the finely structured lunar regolith at cm scales and places tight constraints on geologic processes related to the formation of the swirls. That is, the viability of the dust levitation and comet swarm impact models hinges on the ability to demonstrate that the roughness characteristics of the swirls would not be altered by (1) piling of fine-grained dust, resulting in smoother surfaces at cm scales or (2) regolith disturbance and impact scouring resulting in a layer of fine particulates at cm scales. Figure 6: Reiner Gamma roughness model. Modelled brightness temperature deviations between the channels 3 and 6 as function of the local time are plotted for RMS surface slopes varying in 5° increments from 10° (bottom line) to 40° (top line). Measured data from the Reiner Gamma swirl are displayed as magenta circles. Data from a nearby off-swirl surface are displayed as blue squares. Error bars are 1 s.d. Curves representing 25–30° roughness are bold. Diviner data from Reiner Gamma swirl indicate surface roughness in this range. Full size image Thermophysical characteristics of swirls Diviner night-time data and thermal models can also help to differentiate between the competing formation mechanisms for the lunar swirls. Cooling of the lunar surface throughout the night provides information on the physical nature and degree of processing of the lunar regolith, including rock abundance and vertical structure and particle size of the regolith fines [21] , [22] . We constructed 128-ppd night-time temperature maps using Diviner channel 8 (50–100 μm) brightness temperatures acquired between local times of 19:30 and 05:30 ( Fig. 7 ). Reported values are positive or negative deviations from the scene average normalized for local time variations. On-swirl and off-swirl temperature averages were determined using the same regions of interest shown in the boxes in Fig. 1 . The average normalized temperature on the sampled portion of the Reiner Gamma swirl is −0.8±1.5 K as opposed to the average off-swirl temperature of −0.3±1.8 K (1- σ s.d.). The sampled portion of the swirl, on average, is only ~0.5 K colder than the off-swirl surface, but it is visible in the stretched night-time temperature image (white arrows in Fig. 7a ). 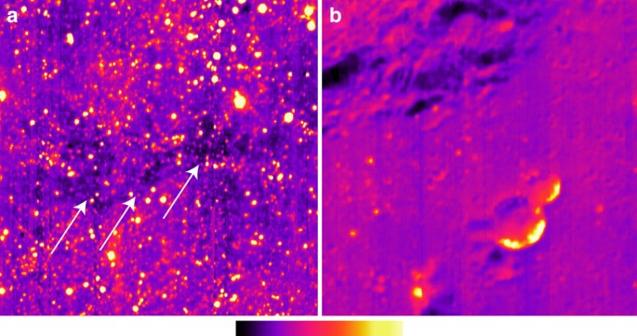Figure 7: Diviner night-time temperature data for the Reiner Gamma and Van de Graaff crater swirls. Area of each image is same as Wide Angle Camera base maps inFig. 1a,b. (a) Average normalized night-time temperature for Reiner Gamma, stretched from −3.6 to 7.0 ΔK. Arrows show the colder temperatures associated with the swirl. (b) Average normalized night-time temperature for Van de Graaff crater, stretched from −7.0 to 15 ΔK. At the Van de Graaff crater site, the average on-swirl normalized night-time temperature is 0.4 K, while the off-swirl average is 0.0 K. Figure 7: Diviner night-time temperature data for the Reiner Gamma and Van de Graaff crater swirls. Area of each image is same as Wide Angle Camera base maps in Fig. 1a,b . ( a ) Average normalized night-time temperature for Reiner Gamma, stretched from −3.6 to 7.0 ΔK. Arrows show the colder temperatures associated with the swirl. ( b ) Average normalized night-time temperature for Van de Graaff crater, stretched from −7.0 to 15 ΔK. Full size image The measured temperature differences, though small, can be tied directly to the physical properties of the swirl surfaces. To do this, we use a thermal model to constrain the differences in regolith properties between the swirl and non-swirl surfaces. This standard lunar regolith model [22] , [38] uses Diviner night-time temperature data to constrain the upper regolith density profile. Using the on- and off-swirl surfaces delineated in Fig. 1a , and the Clementine 750-nm albedos of these regions, we show that the temperature difference between the on- and off-swirl surfaces can be accounted for completely by the albedo difference between the swirls ( Fig. 8 ). In addition, we added a 2-mm low thermal inertia (~30 J m −2 K −1 s −1/2 , ~50% of the standard model) layer on top of the standard swirl model. Such a low thermal inertia layer would be expected from the admixture of additional fine particulates with typical lunar regolith [39] . It is possible, however, that this model does not capture the effects of the minor admixtures of fine particulates with the bulk lunar regolith. Nevertheless, our results show that even this 2-mm thick layer would produce night-time temperatures much lower than those that are observed. Put another way, the swirls are surficial features that, thermophysically, are nearly indistinguishable from the surrounding terrain. The surficial nature of the swirls as determined by Diviner is consistent with Mini-RF radar observations of these features [40] . 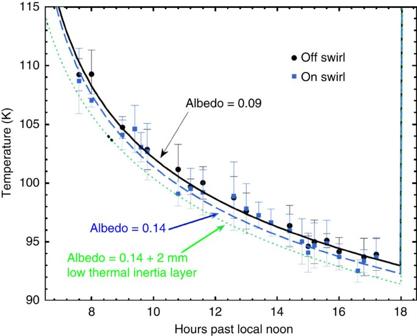Figure 8: Reiner Gamma thermal model. Diviner night-time temperature observations on (blue dots) and off (black dots) the Reiner Gamma swirl are plotted and compared with two thermal models. Error bars indicate standard 1 s.d. in temperature measurements within the spatially binned measurement regions (Fig. 1a). The black solid line and blue dashed line show the predicted temperatures using the standard regolith model21,37. Predicted night-time temperatures for a 2-mm thick low thermal inertia layer on top of the standard swirl thermal model (green dotted line) are too low to explain temperatures observed by Diviner. Figure 8: Reiner Gamma thermal model. Diviner night-time temperature observations on (blue dots) and off (black dots) the Reiner Gamma swirl are plotted and compared with two thermal models. Error bars indicate standard 1 s.d. in temperature measurements within the spatially binned measurement regions ( Fig. 1a ). The black solid line and blue dashed line show the predicted temperatures using the standard regolith model [21] , [37] . Predicted night-time temperatures for a 2-mm thick low thermal inertia layer on top of the standard swirl thermal model (green dotted line) are too low to explain temperatures observed by Diviner. Full size image The lunar regolith has been highly processed by impact gardening that produces a delicate vertical structure with unique thermophysical properties. Any deviation from this structure shows clear night-time temperature differences that are easily identified in Diviner data [21] , [22] , [28] and are absent from the swirl sites. For example, recent impacts by swarms of meteors or comets, [4] , [5] , [6] although they might not produce a 2-mm thick low thermal inertia layer as modelled in Fig. 8 , would almost certainly disturb the regolith vertical structure and lead to clearly observable temperature and roughness phenomena in the Diviner data. Previous spectroscopic observations of the swirls at visible and near-infrared wavelengths have been used to argue for the solar wind standoff model [3] , [14] , [24] , the micrometeoroid/comet swarm model [4] , [5] , [6] or the feldspathic dust pile model. More recently, M 3 spectra have been used to propose a hybrid model for swirl formation that invokes both regolith disturbance and dust lofting [41] . The mid-infrared Diviner data presented here place tight constraints on the swirl formation process and must be accounted for by any proposed swirl formation mechanism. The proposed feldspathic dust lofting [7] , meteoroid/comet swarm [4] , [5] , [6] and hybrid [41] swirl formation mechanisms would likely result in thermophysical and spectral properties that are inconsistent with the Diviner measurements. The proposed dust lofting and hybrid processes cannot account for the observed CF shift in Diviner data while the meteoroid/comet swarm and hybrid processes cause regolith disturbance that would result in a substantial thermal anomaly in the night-time Diviner data. On the other hand, the solar wind standoff mechanism for swirl formation would lead to a slight shift of the CF to shorter wavelengths compared with the surrounding regolith due to a reduction in space weathering, but show no difference in the unique lunar regolith thermophysical properties because impact gardening is otherwise unaffected. These properties are exactly what are observed, and the Diviner observations, in addition to M 3 and Mini-RF [14] , [15] , [40] observations and laboratory experiments [42] , strongly support the solar wind standoff hypothesis for lunar swirl formation. Because they are clearly associated with magnetic field anomalies, lunar swirls present an opportunity to study and isolate the effects of solar wind sputtering/implantation and micrometeoroid bombardment processes on optical maturity. The immature nature of the swirls suggests that solar wind sputtering and implantation, which is prevented by local magnetic fields at the swirl sites, is the primary process for space weathering and optical maturation of airless body surfaces that do not have a global magnetic field, while micrometeoroid bombardment and resulting vapour deposition plays a subordinate role. The results of this study should motivate additional space-weathering experiments and work on the mature lunar regolith samples to test this hypothesis. Diviner CF calculations and average spectra The Diviner Lunar Radiometer Experiment on board the Lunar Reconnaissance Orbiter is an infrared radiometer with two solar reflectance channels and seven channels in the thermal infrared wavelength range, including three narrow band channels that span the wavelength ranges 7.55–8.05 μm, 8.10–8.40 μm and 8.38–8.68 μm. These ‘8 μm’ channels can be used to calculate the position of the silicate CF [17] that is directly sensitive to the degree of silica tetrahedral polymerization and bulk SiO 2 content [18] . By viewing lunar surface targets multiple times under different viewing conditions, the precision of individual Diviner CF values, which are known to be systematically affected by illumination and viewing geometry, are estimated at<0.02 μm (refs 17 , 43 ). For this study, we used data collected between 8:30 and 16:30 local solar time, with emission angles <5 ° from nadir. These restricted ranges minimize the effects of the observation conditions on Diviner CF estimates. All data used in the current study were reduced using the most recent available corrections [44] . CF values were modelled following the methods of Greenhagen et al . [17] In brief, the shapes of the CFs for the regolith surfaces of airless bodies can be approximated as parabolas. Each three-point Diviner spectrum is fit as a parabola by solving the following system of three equations to find the wavelength of the parabola maximum, λ Max : In these equations, y 3 , y 4 and y 5 are the emissivities for Diviner channels 3, 4 and 5, respectively, and A, B and C are constants. The calculated CF value is λ Max . To generate the representative three-point spectra, we averaged groups of 7,897 and 8,181 Diviner spectra to produce representative on-swirl and off-swirl spectra, respectively, at Reiner Gamma and model the CFs for these regions. At the Van de Graaff crater site, we averaged 1,736 spectra each for the on-swirl and off-swirl regions. Thermal model The one-dimensional thermal model employs standard forward difference approximations for spatial and temporal derivatives and incorporates important constraints and improvements based on fits to the Diviner data [22] , [38] . Most important of these are depth-dependent and temperature-dependent thermal conductivity, as well as spatially variable regolith porosity and rock abundance. Model layer thicknesses are typically<1 mm, and the bottom boundary at 2 m is well below the ~10 cm skin depth of the diurnal thermal wave. We allow the model to fully equilibrate over at least 10 years before reporting the results. Roughness model The effects of roughness on thermal emission are simulated using a modified statistical shadowing model similar to several that have previously been described in the literature [29] , [36] , [37] . Using this model, we predicted the surface temperatures for slopes from 0 to 90° and azimuth orientations from 0 to 360°. We then convolved each calculated temperature with its expected fractional surface area for the given RMS slope, based on the assumed Gaussian height distribution [30] . Infrared emission at the given measurement wavelength is then calculated as a weighted sum of the contributions of all the surface elements (both illuminated and shadowed) within the field of view [28] . The model also incorporates a shadow approximation [31] , [33] that accounts for the statistical likelihood of a surface to be within a shadow cast by another surface. Night-time data Night-time (19:30 to 05:30 local time) temperature maps were constructed from the Diviner Level 2 Gridded Data Products available at the Planetary Data System. A total of 46 separate Diviner channel 8 (50–100 μm) brightness temperature maps were assembled from a single Lunar Reconnaissance Orbiter mapping cycle collected over the course of a lunar day. The average brightness temperature was subtracted from each map to normalize the temperature for the local time variations. The normalized maps were averaged to produce the final temperature deviation maps. This methodology ensures that any temperature differences between on swirl and off swirl are preserved. How to cite this article: Glotch, T. D. et al . Formation of lunar swirls by magnetic field standoff of the solar wind. Nat. Commun. 6:6189 doi: 10.1038/ncomms7189 (2015).